Picometre-precision analysis of scanning transmission electron microscopy images of platinum nanocatalysts Measuring picometre-scale shifts in the positions of individual atoms in materials provides new insight into the structure of surfaces, defects and interfaces that influence a broad variety of materials’ behaviour. Here we demonstrate sub-picometre precision measurements of atom positions in aberration-corrected Z-contrast scanning transmission electron microscopy images based on the non-rigid registration and averaging of an image series. Non-rigid registration achieves five to seven times better precision than previous methods. Non-rigidly registered images of a silica-supported platinum nanocatalyst show pm-scale contraction of atoms at a ( )/( ) corner towards the particle centre and expansion of a flat ( ) facet. Sub-picometre precision and standardless atom counting with <1 atom uncertainty in the same scanning transmission electron microscopy image provide new insight into the three-dimensional atomic structure of catalyst nanoparticle surfaces, which contain the active sites controlling catalytic reactions. Nanometre-scale, heterogeneous objects often depend on their surfaces for important properties and function; however, solving such structures is difficult enough to have earned the name ‘the nanostructure problem’ [1] . Nanocatalysts, such as platinum (Pt) nanoparticles (NPs), are a prototypical example of the nanostructure problem [2] , since their morphology and especially the detailed atomic structure of their surfaces is crucial to their catalytic activity [3] , [4] , [5] , [6] . Transmission electron microscopy (TEM) and scanning TEM (STEM) have been used nearly since their inception for NP characterization but have been limited by the available resolution and precision [7] , [8] , [9] , [10] . Aberration correction has made sub-Angstrom spatial resolution routine in TEM and STEM. Once atoms can be resolved, the question becomes how precisely can their positions be measured. (Resolution is the smallest distance between two objects in an image at which the objects appear distinct. Precision is the statistical spread of repeated distance measurements in an image.) Precision smaller than the resolution is routinely achievable [11] , [12] , [13] , [14] : the best reported precision for TEM and STEM images is 1–3 picometre (pm) (refs 11 , 12 ) and 4–5 pm (refs 13 , 14 ), respectively. Precision is fundamentally limited by the signal-to-noise ratio (SNR) [15] ; however, in STEM serial acquisition of pixels translates instabilities in the sample and probe positions into displacements of the imaged atoms, limiting precision well above the SNR limit. Averaging many frames can reduce instabilities and increase SNR [11] , [13] ; however before averaging, the frames must be registered to one another to account for, for example, drift of the sample between frames. Here we develop a non-rigid (NR) registration scheme that enables us to achieve extremely high SNR images. We demonstrate sub-picometre (pm) precision measurements of atom positions in aberration-corrected Z-contrast STEM images, more than five times better than previous methods [13] , [14] , based on NR registration and averaging of an image series. NR registered images of a Pt nanocatalyst show pm-scale contraction of atoms at a ( )/( ) corner towards the particle centre and expansion of a ( ) facet. Combined with standardless atom counting [16] to determine three-dimensional (3D) structure, sub-pm precision STEM can give new insight into the active sites controlling catalytic reactions, and the displacements from defects, interfaces or various ferroic phenomena. Non-rigid registration Registering two images, R and T , requires finding a deformation phi of the image domain such that the composition T ○ phi agrees with R . 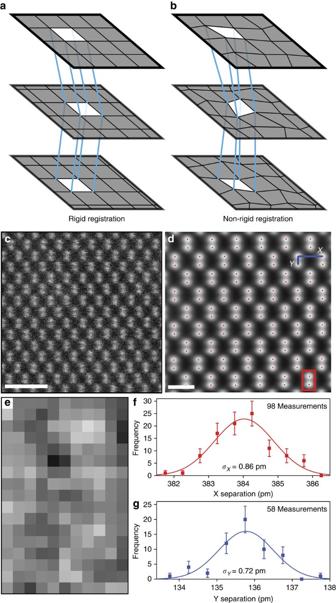Figure 1: Sub-pm precision STEM imaging with NR registration. Diagrams showing (a) rigid and (b) NR registration of an image series without and with distortions, respectively. (c) The first raw HAADF STEM image of the Si [110] series. The scale bar is 1 nm. (d) The average image after the NR registration. The red markers indicate the series-averaged atomic column positions determined from fitting. The scale bar is 400 pm. (e) The residual of a two 2D Gaussian fit to the Si dumbbell in the red box ind. The maximum intensity in the residual is 0.5% of the column peak intensity. (f,g) Histograms of the measured separations between the atomic column positions in thexandydirections defined by the blue axes ind. The error bars in (f) and (g) are the square root of the frequency and the curves are the best-fit normal distributions. Figure 1a shows the conventional approach, in which phi is a rigid translation [11] , [13] , [14] . A rigid phi works for the unchanging pixel grid in Fig. 1a , but it can lead to a loss of resolution and precision if there are distortions from serial acquisition, as shown in Fig. 1b . Our NR registration scheme uses a pixelwise, non-parametric deformation phi NR , which can account for all sources of image distortion including probe instabilities and sample drift. Figure 1: Sub-pm precision STEM imaging with NR registration. Diagrams showing ( a ) rigid and ( b ) NR registration of an image series without and with distortions, respectively. ( c ) The first raw HAADF STEM image of the Si [110] series. The scale bar is 1 nm. ( d ) The average image after the NR registration. The red markers indicate the series-averaged atomic column positions determined from fitting. The scale bar is 400 pm. ( e ) The residual of a two 2D Gaussian fit to the Si dumbbell in the red box in d . The maximum intensity in the residual is 0.5% of the column peak intensity. ( f , g ) Histograms of the measured separations between the atomic column positions in the x and y directions defined by the blue axes in d . The error bars in ( f ) and ( g ) are the square root of the frequency and the curves are the best-fit normal distributions. Full size image Estimating phi NR is an underconstrained problem. Our solution is summarized here and described in greater detail in the Supplementary Methods and elsewhere [17] . We employ a variational approach to minimize the sum of the negative normalized cross correlation, E NCC , of T ○ phi NR and R , and the Dirichlet energy of the displacement, as a regularizer on phi NR . Thus, we seek to minimize where λ is a non-negative, constant parameter that controls the smoothness of the deformation, Ω is the image domain, Ω is the Jacobian of phi and 1 is the identity matrix. To avoid being trapped by local minima in E [ phi NR ] for nearly periodic STEM images, we use a coarse-to-fine multilevel approach. It initially registers down-sampled variants of the images, and then uses the resulting phi NR as an initial guess at the next finer sampling levels, iterating up to the original sampling. At each level, we solve the minimization problem by relating it to a time-dependent partial differential equation and using a regularized gradient descent [18] with explicit time discretization and step size control [19] . To register the entire sequence of images T 0 , …, T N , we first find the NR deformations phi j+ 1 ,j between all pairs T j and T j +1 , and then register the entire series to T 0 using phi j +1 , j ○ phi j ,0 as the initial guess for phi j +1,0 . Then, we repeat the registration using the average of the registered frames as the reference frame and iterate to find the final set of deformations. The NR registration technique makes some assumptions about the imaging process (discussed in the Supplementary Methods ) but no assumptions about the object. In principle, any technique subject to pixel distortions can benefit from NR registration, including cryo-TEM and atomic force, scanning tunnelling or scanning electron microscopy. The NR registration software is available by request to the authors. Sub-pm precision on single crystal materials Figure 1c–g demonstrates that NR registration of aberration-corrected STEM images achieves sub-pm precision. Experimental details are in the Methods section and in Supplementary Note 1 . Figure 1c shows the first image of a 512-high-angle annular dark-field (HAADF) STEM image series of silicon (Si) [110]. The image series was averaged after NR registration to create the final HAADF image in Fig. 1d , which therefore shows the average sample structure over the image series acquisition time. Owing to the long acquisition time of the averaged image, fast processes such as thermal displacements and atom displacements from electron beam momentum transfer are not captured. The entire series is shown raw in Supplementary Movie 1 and registered in Supplementary Movie 2 . Typical NR pixel deformations for one image in the series are shown in Supplementary Fig. 1 and discussed in Supplementary Note 1 . Distortions from circular symmetry in the Si atomic columns in Fig. 1d are likely due to residual lower-order aberrations in the electron probe. Each Si dumbbell was fit to the sum of two, two-dimensional (2D) Gaussian functions to find the series-averaged atomic column positions. Figure 1e shows a typical featureless fit residual. Figure 1f,g shows histograms of the 98 and 58 measured x and y Si column separations, respectively, defined in Fig. 1d . Following Bals et al. [11] , we define the precision σ of the image as the standard deviation (s.d.) of these separations; therefore, σ x =0.86 pm and σ y =0.72 pm. Another measure of image precision is the uncertainty in the atom column’s fit position [20] , which yields σ x =0.36 pm and σ y =0.60 pm, again sub-pm. A similar experiment showing sub-pm precision for gallium nitride (GaN) is shown in Supplementary Fig. 2 and Supplementary Movies 3 and 4 , and discussed in Supplementary Note 2 . Supplementary Fig. 3 and Supplementary Note 3 show that rigid registration of the same Si HAADF image series results in precisions of σ x =5.3 pm and σ y =4.0 pm, five to seven times larger than NR registration. NR registration is further validated using simulated STEM distortions, including preservation of inhomogeneous strain fields with pm precision, as shown in Supplementary Fig. 4 and Supplementary Movie 5 , and discussed in Supplementary Note 4 . Supplementary Figs 5 and 6 and Supplementary Note 5 show how NR registration enables the tracking of image precision, resolution, sample damage and focus drift, as a function of time and electron dose through the STEM time series. Reproducible, sub-pm precision imaging enables measurement of lattice strains <1% associated with defects and interfaces, ion displacements associated with ferroic behaviour, and relaxation at surfaces, all with the well-established interpretability, quantifiability and analytical capability of STEM. 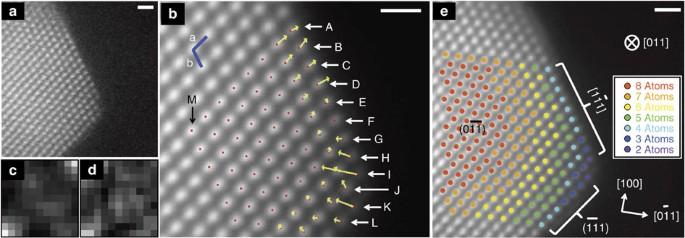Figure 2: Pt nanocatalyst surface atom displacements and 3D structure. (a) The first raw HAADF STEM image of the [011] Pt nanocatalyst series. (b) The average image after NR registration. The red markers are the series-averaged atomic column positions determined from fitting, and the yellow arrows are magnified atom column displacement vectors. The displacement magnitudes of the labelled atoms inbare given inTable 1. (c,d) The fit residuals for the columns M and I, respectively, inb. The maximum intensity incis 2.8% of the column peak intensity due to slight overlap with a neighbouring atom column. (e) The number of atoms in each column determined by comparing the experimental absolute intensities to simulations. All scale bars are 500 pm. Platinum nanocatalyst structure Figure 2 shows results from a HAADF STEM image series of a 6.5-nm diameter Pt catalyst NP along [011] on a silica support. Experimental details are in the Methods section and in Supplementary Note 6 , and the entire series is shown raw in Supplementary Movie 6 and registered in Supplementary Movie 7 . Figure 2a shows the first HAADF STEM image in the series. The first 56 images in the series were NR-registered and averaged to create the final HAADF image in Fig. 2b . Series-averaged atomic column positions were determined by fitting to a 2D Gaussian function. Figure 2c,d show representative fit residuals of one interior and one surface column, marked by M and I, respectively. They show some diagonal structures probably due to residual aberrations such as astigmatism. Analysis of 53 Pt atom columns at least five atomic planes from the surface yielded σ a =2.5 pm and σ b =1.3 pm for the a and b separations defined in Fig. 2b . The reduced precision results from decreased SNR due to the lower dose required to avoid damage and the lower scattering power of the small NP. The fit position uncertainties are σ x =1.5 pm and σ y =1.6 pm, indicating that the instability and SNR precision limits are similar. The fit uncertainty is used as the displacement uncertainty for surface atoms, as discussed in the Methods section. Figure 2: Pt nanocatalyst surface atom displacements and 3D structure. ( a ) The first raw HAADF STEM image of the [011] Pt nanocatalyst series. ( b ) The average image after NR registration. The red markers are the series-averaged atomic column positions determined from fitting, and the yellow arrows are magnified atom column displacement vectors. The displacement magnitudes of the labelled atoms in b are given in Table 1 . ( c , d ) The fit residuals for the columns M and I, respectively, in b . The maximum intensity in c is 2.8% of the column peak intensity due to slight overlap with a neighbouring atom column. ( e ) The number of atoms in each column determined by comparing the experimental absolute intensities to simulations. All scale bars are 500 pm. Full size image Figure 2b shows the displacement of surface Pt atoms with respect to the atomic lattice of the particle interior. The displacement magnitudes of the labelled columns are given in Table 1 . As STEM images are a 2D projection, we cannot extract the [011] component of the atom displacements. Within this limitation, columns A–D show bond length expansion away from the NP centre along [ ], while columns G–L show bond length contraction towards the NP centre along [ ]. All the uncertainties for atom columns A–D and G–L are smaller than the measured displacements. E and F are transition columns between contraction (G–L) and expansion (A–D); therefore, the uncertainties are similar to the smaller displacements. The corner column I shows the largest bond length contraction of 18.5±4.1%. Column D shows the largest expansion of 6.4±1.1%. Table 1 Pt nanocatalyst surface atom displacement magnitudes. Full size table Figure 2e shows the number of atoms in each Pt column, determined following LeBeau et al. [16] by comparing the absolute experimental intensity to simulations as described in the Methods section, Supplementary Fig. 7 and Supplementary Note 8 . This area of the NP has one to eight atoms per Pt column. Variability in the support scattering is a larger contribution to the uncertainty in the number of atoms in each column than the Poisson noise, unlike previous work that was SNR-limited [16] . The image contrast just outside the NP may also indicate the presence of surface hydrocarbons or oxygen, another limitation to quantification that is not considered in simulations. Primarily due to support scattering variability, ~40% of the atoms could have either one more or one less atom than shown in Fig. 2e , but the assignments for the other ~60% are unique. NR registration yields a moderate improvement over rigid registration for standardless atom counting for this data set, as shown in Supplementary Fig. 8 and discussed in Supplementary Note 8 . The well-defined terraces and monatomic steps arose naturally from the quantification. The NP has two {111} surfaces on the right side out of the image plane that are four atoms thick and thin to two atoms thick near the ( )/( ) corner. There is a correlation between lattice contraction and lower number of atoms in the column, like near the corner, and lattice expansion and larger number of atoms in the column, like near the surface facet. On the left, there is a flat ( ) surface facet in a region eight atoms thick. We cannot distinguish surface steps on the NP top and bottom surfaces experimentally, but if we assume that the metal–support interaction results in a flat (011) plane against the silica support [21] , then the particle consists of one- to two-atom wide ( ) terraces with monatomic ( ) and ( ) steps propagating from the out-of-plane ( ) and ( ) facets to the in-plane ( ) facet. The edges that create this terraced structure generally run parallel to the ( ) and ( ) surface facets. There is intensity consistent with one atom at the very tip of the NP corner between atoms I and K, but it does not form a peak distinct enough for fitting. We speculate that there was an atom at the corner, but it experienced large motions near its lattice site during acquisition. It cannot have been displaced from the particle by the electron beam during the series, or the intensity would be less than one atom. In the future, modelling atom vibrations at surfaces under the influence of the electron beam will be required to extract the maximum possible information from low-noise, low-distortion STEM images. Observations of average bond contraction at flat metal surfaces [22] , [23] can be explained by the lower coordination of surface atoms [24] or the electrostatic force from surface rearrangements of the electronic charge [25] , [26] . Both explanations predict a larger bond contraction of corner atoms near facet edges and steps, consistent with our observation of bond length contraction near the NP tip. However, the varying magnitude and direction of the contraction, and the observed expansion along the ( ) surface facet, emphasize the need for detailed microscopic investigations of real, 3D structures, not just idealized 2D surfaces. Our results agree with previous microscopic investigations on some points, but not others. Comparable measurements have been made on Pt nanocatalysts on a carbon support by Chang et al. [10] using TEM and on faceted Au NPs dispersed on graphene by Huang et al. [27] using coherent electron nanodiffraction. The bond length contraction near the corner in Fig. 2b is in reasonable agreement with Huang’s report of 22-pm contraction of edge and corner bonds but is in disagreement with Chang’s report of 14–30-pm bond length expansion of a similar (110)−(1 × 1) reconstructed ( )/( ) corner. However, Chang also reports density functional theory (DFT) calculations that predict the contraction of a (110)−(1 × 1) reconstructed ( )/( ) corner [10] , in reasonable agreement with our results. We report expansion of a ( ) surface, as does Chang, but Huang reports only contraction. We report displacements primarily along the vectors pointing to the particle centre (along [ ] for ( )/( ) corner atoms and along [ ] for ( ) surface atoms) and very little lateral displacements. Chang et al. [10] reports significant lateral displacements along the surface at microfacet risers, which are not present on our NP. Adding high-precision STEM as a new imaging modality capable of quantitatively addressing these problems will stimulate further research to identify the reliable measurements and resolve these discrepancies. In conclusion, sub-pm precision measurement of the positions of atoms has been achieved in STEM by NR registration and averaging of a series of short-exposure images. Picometre precision makes it possible to measure the small but crucial atomic displacements typical for surfaces, interfaces, defects and ferroic phenomena. Using this method, we have measured pm-scale bond length variations at the surface of a Pt nanocatalyst, showing large bond length contraction at a ( )/( ) corner but significant expansion along a ( ) surface. NR registration also enables standardless atom counting without limitation by Poisson noise, which elucidates the 3D structure of the nanocatalyst with <1 atom uncertainty. High-precision measurements of nanocatalyst surfaces may enable new insight into the correlation between structure and catalytic function. HAADF STEM experiments All atomic-resolution STEM experiments were performed on a FEI Titan microscope equipped with a CEOS probe aberration corrector operated at 200 keV. HAADF STEM images were collected with a 24.5-mrad probe semi-angle, 24.5-pA probe current, STEM resolution of ~0.9 Å and HAADF detector range of 54–270 mrad. In this imaging mode, the atomic column intensity is approximately proportional to Z 1.7 , where Z is the atomic number of the atoms under the electron beam. Each STEM series was acquired with known HAADF detector gain and probe current, so the data can be placed on an absolute intensity scale [28] , [29] . The STEM probe current was measured on the Titan’s Gatan US1000 CCD camera, which has known gain from prior calibration. The Fischione HAADF detector black level was measured from an image with the beam blanked, and the gain was measured from an image acquired with the full STEM probe on the detector. By collecting these experimental parameters during each experiment, the HAADF image intensity can be converted to the number of collected electrons per pixel, as required to estimate the Poisson noise, or put on a fractional absolute intensity scale relative to the incident beam intensity, as required for quantitative comparison with HAADF image simulations. Electron-transparent STEM samples of single crystal diamond cubic Si and wurtzite GaN were created by wedge-polishing followed by final thinning in a Fischione 1010 ion mill. Before STEM experiments, samples were plasma-cleaned in a Fischione plasma cleaner in a 75% argon–25% oxygen mixture for 5 min to eliminate organic carbon surface contamination. Si was imaged along [110], producing dumbbells of Si columns with a dumbbell separation of 1.36 Å. As a result of the Z -contrast nature of HAADF STEM images and the atomic number difference of Ga and N, atomic-resolution imaging of GaN along results in invisible N atomic columns and visible Ga atomic columns with a projected nearest neighbour separation of 2.76 Å. The Pt NP catalysis sample was created by impregnating amorphous silica with a total of 0.35% Pt followed by a heat treatment at 525 °C as described by Jackson et al. [30] , resulting in 1- to 7-nm Pt NPs scattered on a silica support. The STEM sample was prepared by dispersing this catalysis material on a lacey carbon TEM grid. A face-centred cubic crystalline Pt NP was imaged along [011], producing Pt columns with a projected separation of 2.40 Å. HAADF STEM image simulations Frozen phonon multislice simulations as implemented by Kirkland [31] were used for the standardless atom counting of the Pt nanocatalyst, the source size determination using GaN data and the Si dislocation distorted image series analysis. At 300 K, the root-mean-square displacements of Si, Ga and Pt atoms in the structures we studied are 0.076, 0.060 and 0.067 Å, respectively [32] , [33] , [34] , [35] . Images of a Pt [011] atom column of varying thickness were calculated using 160-phonon configurations. The Pt [011] crystal was 33 Å × 31 Å and was sampled with a 2,048 × 2,048 pixel wavefunction so the experimental detector angles could be used. The same crystal size and sampling was used for the GaN calculations. The simulated images were convolved with the 88.2-pm full-width at half-maximum (FWHM) Gaussian function to account for incoherent source broadening [28] , and then the average simulated intensity was calculated from a window with the same size that was used in the experimental intensity analysis, centred on the simulated Pt column, as a function of thickness. An image of a Si [110]-dislocation model was calculated using 16-phonon configurations. A 100 Å × 103 Å × 76 Å segment of the molecular dynamics model with one dislocation was extracted for the STEM simulation, which used a 2,048 × 2,048 pixel wavefunction. A 512 pixel × 512 pixel, 78 Å × 78 Å image with the dislocation core at the centre was calculated with the pixel size chosen to match the experimental Si data set in Fig. 1 . Limited reciprocal space sampling required detector angles of 54–150 mrad, instead of 54–270 mrad, as used in experiments. The simulated image was convolved with the 88.2-pm FWHM Gaussian function to account for incoherent source broadening. Incoherent source broadening measurement Quantitative matching between STEM simulations and experiments requires accounting for the incoherent source broadening in the image [36] , [37] . Following LeBeau et al. [28] , [29] , we adopt a Gaussian source, although other source functions have been investigated [37] . The FWHM of the Gaussian was determined for the UW-Madison Titan microscope by minimizing the χ 2 between a single experimental HAADF STEM image of GaN and frozen phonon multislice simulations as a function of the diameter of the Gaussian source function. An experimental PACBED pattern acquired at the same location as the experimental HAADF STEM image was compared with frozen phonon multislice-simulated PACBED patterns to determine the experimental sample thickness [38] . The best-fit FWHM was 88.2 pm, consistent with previous reports on similar microscopes [28] , [29] . Fitting precision and displacement analysis Owing to sample drift during image series acquisition, only a sub-area of the whole averaged image uses all the images in the series for the average. Only that area was used for further analysis. To achieve sub-pixel location of the atomic column positions, we fit a small region of pixels around each atomic column to a 2D Gaussian function plus a constant, using the standard Levenberg–Marquart L 2 -norm minimization method. The fit parameters are I 0 , A , x w , y w , x 0 , y 0 and c , and x and y are the positions for the intensity I . For the Si images, each dumbbell was fit to the sum of two 2D Gaussian functions to fit both atom columns in the dumbbell at the same time. For the GaN and Pt images, each Ga and Pt column was fit to a single 2D Gaussian function. As discussed in the previous section, the shape of the column images is dominated by the incoherent source broadening, which is well-approximated by a Gaussian. The number of pixels around each column and the position of the fit window was optimized to achieve the best-fit to Equation 2, defined as the fit with the lowest χ 2 . Each fit was weighted by the Poisson noise (square root of the total number of electrons, , detected in each pixel of the averaged image) in order to estimate the uncertainties in the fit parameters. The s.d. of a single pixel through the registered image series [20] for a pixel inside a Si [110] column is 3.6 e − , while =10.6 e − for the same pixel. Therefore. using to weight the fits is a conservative estimate of the noise and thus of the fit parameter uncertainties. This result also shows that other forms of noise, such as detector noise, are small. The reduced noise in the registered series is most likely a result of the bilinear interpolation step used to apply sub-pixel shifts from the NR registration. Once atom column locations were found for the Si and GaN images, the separations between the columns in the x and y directions (indicated by the blue axes in each image set) were calculated. The average x and y separations were used to calibrate each image’s spatial pixel size to the known atomic structure independently in x and y . This spatial calibration corrects for the ~1% pixel non-squareness in the scan. As the a and b axes in the Pt image series do not correlate to the x and y scan directions, the image was spatially calibrated in the x and y directions using the average of the average a and b separations from an interior area of the NP. Two measures of precision ( σ ) were used: (1) the s.d. in the measured x and y separations for Si and GaN, and a and b separations for the Pt data, and (2) the average fit uncertainty in locating the atom column position relative to the scan x and y directions. As the scan direction correlates to the x and y blue axes for GaN and Si, both definitions measure the precision in the same direction. As the scan direction does not correlate to the a and b blue axes for Pt, the two precision definitions measure the precision in different directions. The images in all figures have not been rotated, so the horizontal and vertical directions are the scan x and y directions, respectively. For the Pt image series, the image area at least five atomic planes from the surfaces in projection was used to calculate the precision to avoid the effect of surface atom bond length variation on the s.d. of the measured interatomic column separations. For the Pt particle, we constructed a perfect reference lattice to measure surface displacements by measuring the average a and b lattice parameters from the image area used for precision analysis, and then aligning the reference lattice to the image by minimizing the root-mean-squared displacement between the positions of the reference lattice and the atomic columns. The average displacement between the positions of the reference lattice and the fit positions in the precision calculation area is 2.0 pm, consistent with the measured precision from this area. The surface atom displacements are the vector difference between the measured position and the closest point on the reference lattice. The uncertainties in the displacements are the average of the x and y fit position uncertainties weighted by the angle of the displacement vector. Molecular dynamics simulations NR registration is validated using simulated images of a Si dislocation core as a test sample, as shown in Supplementary Fig. 4 and discussed in Supplementary Note 4 . Molecular dynamics simulations implemented in the Large Scale Molecular Dynamics Simulator (LAMMPS) software (at http://lammps.sandia.gov/ ) using the Tersoff potential [39] were used to determine the structure of the Si dislocation core. The cohesive energy of a Si single crystal was calculated to be 4.61 eV, in a good agreement with published experimental values (4.55–4.90 eV) [40] . Dislocations were modelled in a 66,420-atom cell with dimensions 16.1 nm × 21.7 nm × 3.8 nm along the x =[110], y =[ ] and z =[ ] directions, respectively. A dislocation dipole consisting of two perfect edge dislocations of the opposite sign and with dislocation lines being parallel to the z axis were modelled. Periodic boundary conditions were applied in all three spatial directions, and the system size was large enough so that the overlap of strain fields from periodic images of dislocations was negligible. The system was relaxed at 5 K and zero pressure in a constant pressure-constant temperature ensemble using a Nose Hoover thermostat and barostat. The resulting structure of the dislocation core is in agreement with published structures generated using molecular dynamics [41] . How to cite this article: Yankovich, A. B. et al. Picometre-precision analysis of scanning transmission electron microscopy images of platinum nanocatalysts. Nat. Commun. 5:4155 doi: 10.1038/ncomms5155 (2014).